CRL4ACRBNE3 ubiquitin ligase restricts BK channel activity and prevents epileptogenesis Ion channels regulate membrane excitation, and mutations of ion channels often cause serious neurological disorders including epilepsy. Compared with extensive analyses of channel protein structure and function, much less is known about the fine tuning of channel activity by post-translational modification. Here we report that the large conductance, Ca 2+ - and voltage-activated K + (BK) channels are targeted by the E3 ubiquitin ligase CRL4A CRBN for polyubiquitination and retained in the endoplasmic reticulum (ER). Inactivation of CRL4A CRBN releases deubiquitinated BK channels from the ER to the plasma membrane, leading to markedly enhanced channel activity. Mice with CRL4A CRBN mutation in the brain or treated with a CRL4A CRBN inhibitor are very sensitive to seizure induction, which can be attenuated by blocking BK channels. Finally, the mutant mice develop spontaneous epilepsy when aged. Therefore, ubiquitination of BK channels before their cell surface expression is an important step to prevent systemic neuronal excitability and epileptogenesis. The activity and expression of ion channels at the cell membrane have to be tightly regulated to maintain ion and fluid homeostasis. Genetic mutations, especially those in genes encoding subunits of voltage-gated and ligand-gated ion channels including BK channels, often alter channel functions and induce epilepsy [1] , [2] , one of the most common chronic neurological disorders found in people of all ages [3] . BK channels are formed by four α subunits [4] and regulated by four types of β subunits in various tissues [5] . It is uniquely activated by both membrane depolarization and increased intracellular Ca 2+ levels [6] , thereby functioning as a neuronal calcium sensor and regulating neurotransmitter release and neuronal excitability [7] , [8] , [9] , [10] . Gain-of-function mutations in BK channel pore-forming α subunit [11] or deletion of the regulatory β4 subunit [12] can lead to enhanced channel activation and development of epilepsy in patients. BK channel function can also be regulated by post-translational modifications such as protein phosphorylation [13] and palmitoylation [14] ; however, the in vivo significance has not been defined. BK channel can interact with CRBN [15] . CRBN was reported to function as a substrate receptor protein for the CRL4A E3 ubiquitin ligase complex composed of DDB1, Cul4A and Roc1 (refs 16 , 17 ); however, substrates targeted by the CRL4A CRBN ubiquitin ligase have not been uncovered. Thalidomide, a small molecule drug approved for treating leprosy and multiple myeloma [18] , directly binds CRBN and inhibits or alters the substrate specificity of the E3 ligase activity of CRL4A CRBN , thus providing mechanistic insight into thalidomide-induced teratogenicity [17] , [19] , [20] . A short carboxyl truncation of CRBN was found in a family with non-syndromic mental retardation [21] , implicating a putative role of CRBN in regulating neuronal activities. Indeed, mice ablated of CRBN show defects in memory and learning [22] . We previously show that DDB1, an essential subunit of the E3 ligase, is critical for survival of neuronal progenitor cells in mouse brain but is likely dispensable for survival of postmitotic neurons [23] . We now generated mice with postnatal deletion of DDB1 in the brain and found that these mice are very sensitive to epilepsy induction and develop spontaneous seizures when they age. We therefore hypothesized that BK channels are substrates of the CRL4A CRBN ubiquitin ligase and the ubiquitination of BK channels is critical for blocking the onset of epilepsy. In the present study, we use pharmacological and genetic approaches to demonstrate that BK channels ubiquitinated by CRL4A CRBN are retained in the endoplasmic reticulum (ER) and prevented from expression at the cell surface. Deregulation of this control mechanism results in enhanced activity of BK channels in cells and epilepsy development in animals. Our finding provides a paradigm for investigating the fine tuning of ion channel activation by protein ubiquitination, particularly in response to pathological insults. CRBN bridges the interaction of BK channels with CRL4A BK channels are tetramers consisting of four α subunits (also called Slo1), each subunit containing seven transmembrane domains and a long carboxyl (C) terminal tail located in the cytoplasm [24] . To identify the interaction domain of Slo1 with CRBN, we first constructed various Slo1 truncations ( Fig. 1a ). The full length or cytoplasmic C terminus, but not the membrane-spanning amino (N) terminus, of Slo1 interacts with CRBN as shown using co-immunoprecipitation assays ( Supplementary Fig. 1a,b ). Both RCK1 and RCK2 domains in the C terminus [25] bind CRBN, and the linker region between these two domains is not involved in the interaction ( Fig. 1b ). Conversely, with a series of CRBN truncations ( Fig. 1c ), the region spanning 81–186 amino acids at the beginning of a putative Lon protease domain and RGS domain in CRBN was found to interact with Slo1 ( Fig. 1d ). 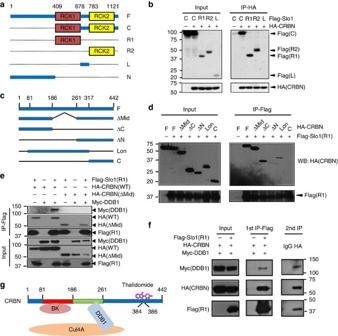Figure 1: BK channels form complexes with CRL4ACRBNE3 ligase. (a) Schematic representation of Slo1 constructs. (b) HEK 293T cells were co-transfected with vectors encoding CRBN together with Flag–Slo1 C (cytoplasmic domain) or its deletion mutants. Protein extracts were subjected to co-immunoprecipitation assay. (c) CRBN constructs are illustrated. (d) HEK 293T cells were transfected with Slo1(R1) vectors together with HA-CRBN or its different truncations. Protein extracts were immunoprecipitated using Flag M2 beads. (e) Vectors encoding Flag-Slo1(R1), Myc-DDB1 and HA-CRBN or HA-CRBN(ΔMid), as a control, were transfected into HEK 293T cells. Protein extracts were immunoprecipitated using Flag M2 beads. (f) HEK 293T cells were transfected with Flag-Slo1, HA-CRBN and Myc-DDB1. Two-step co-IP was performed by initially using Flag M2 beads, followed by elution with the Flag peptide. The eluates were subjected to a second round of IP with anti-HA or control IgG, and the final precipitated proteins were analysed with immunoblotting. (g) Schematic representation of the complex of BK channels with CRL4ACRBNE3 ligase. Figure 1: BK channels form complexes with CRL4A CRBN E3 ligase. ( a ) Schematic representation of Slo1 constructs. ( b ) HEK 293T cells were co-transfected with vectors encoding CRBN together with Flag–Slo1 C (cytoplasmic domain) or its deletion mutants. Protein extracts were subjected to co-immunoprecipitation assay. ( c ) CRBN constructs are illustrated. ( d ) HEK 293T cells were transfected with Slo1(R1) vectors together with HA-CRBN or its different truncations. Protein extracts were immunoprecipitated using Flag M2 beads. ( e ) Vectors encoding Flag-Slo1(R1), Myc-DDB1 and HA-CRBN or HA-CRBN(ΔMid), as a control, were transfected into HEK 293T cells. Protein extracts were immunoprecipitated using Flag M2 beads. ( f ) HEK 293T cells were transfected with Flag-Slo1, HA-CRBN and Myc-DDB1. Two-step co-IP was performed by initially using Flag M2 beads, followed by elution with the Flag peptide. The eluates were subjected to a second round of IP with anti-HA or control IgG, and the final precipitated proteins were analysed with immunoblotting. ( g ) Schematic representation of the complex of BK channels with CRL4A CRBN E3 ligase. Full size image CRBN was co-purified with the CRL4A E3 ubiquitin complex [16] and also identified in our yeast-two-hybrid screening for DDB1-interacting proteins (data not shown). CRBN functions as an adaptor protein for CRL4A E3 ligase, and the CRL4A CRBN is a target of thalidomide-induced teratogenicity [17] . We therefore examined the association between BK channels and the CRL4A CRBN complex. BK channels were found to interact with DDB1 and Cul4A ( Fig. 1e and Supplementary Fig. 1c–e ). CRBN(ΔMid), a truncation mutant ( Fig. 1c ) defective in binding DDB1 (ref. 17 ), still associated with BK channels but failed to mediate the interaction between BK channels and DDB1 ( Fig. 1e ). We further purified the complex by two-step pull-down and elution assays, using lysates from cells co-expressing Flag-Slo1, HA-CRBN and Myc-DDB1. All the three subunits were detected in the final immunoprecipitate ( Fig. 1f ). Endogenous BK channels in the native complex with Cul4A were further confirmed using mouse brain lysates ( Supplementary Fig. 1f ). We conclude that BK channels form complexes with CRL4A CRBN and CRBN bridges the interaction of CRBN with DDB1 and with Slo1 using distinct regions ( Fig. 1g ). CRL4A CRBN targets BK channels for ubiquitination To determine whether BK channels are ubiquitinated by CRL4A CRBN , we performed the following four assays. First, ectopically expressed BK channels co-immunoprecipitated with a high molecular weight ubiquitin smear, and vice versa , suggesting that BK channels are ubiquitinated in these cells ( Fig. 2a ). In addition, only CRBN-interacting regions of Slo1 are ubiquitinated, suggesting that CRBN–Slo1 interaction is a prerequisite for this post-translational modification ( Fig. 2b ). Second, knockdown of endogenous Cul4A, DDB1 or CRBN, but not Cul4B, with small-interfering RNAs (siRNAs) significantly decreased BK channel ubiquitination ( Fig. 2c ). Likewise, the ubiquitination of BK channels was enhanced by the overexpression of Cul4A, DDB1 and CRBN, but not Cul4B ( Supplementary Fig. 2a ). Third, expression of CRBN (ΔMid) markedly decreased BK channel ubiquitination ( Fig. 2d ), consistent with the loss of BK channel interaction with CRL4A ligase ( Fig. 1e ). Finally, BK channel ubiquitination was inhibited by treating cells with thalidomide, a small molecule that directly binds CRBN and inhibits the ubiquitin ligase activity of CRL4A CRBN [17] , or with MLN4924, another small molecule inhibitor of NEDD8-activating enzyme [26] and thereby activities of all Cullin family ligases including CRL4A CRBN ( Fig. 2e and Supplementary Fig. 2b,c ). Taken together, these data indicate that CRL4A CRBN E3 ligase targets BK channels for ubiquitination in cultured cells. 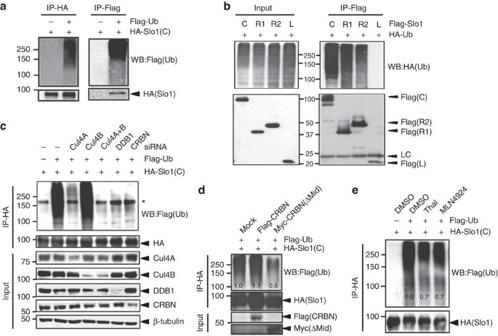Figure 2: CRL4ACRBNtargets BK channels for ubiquitination. (a) HEK 293T cells were transfected with HA-Slo1(C) and Flag-Ub expression vectors. Protein extracts were subjected to co-immunoprecipitation (co-IP) and ubiquitination assays. Ub, ubiquitin. (b) HEK 293T cells were transfected with indicated expression vectors and protein extracts were immunoprecipitated using Flag M2 beads. (c) Effects on BK channel ubiquitination by siRNA knockdown of individual CRL4ACRBNcomplex component. Cul4B is included as a negative control. The star indicates the nonspecific bands. (d,e) Effects on BK channel ubiquitination by (d) overexpression of CRBN(ΔMid), or (e) treating cells with thalidomide (50 μM) or MLN4924 (0.1 μM) for 6 h. Numerical band intensity was measured by NIH Image J and indicated on the figure. Thal, thalidomide. Figure 2: CRL4A CRBN targets BK channels for ubiquitination. ( a ) HEK 293T cells were transfected with HA-Slo1(C) and Flag-Ub expression vectors. Protein extracts were subjected to co-immunoprecipitation (co-IP) and ubiquitination assays. Ub, ubiquitin. ( b ) HEK 293T cells were transfected with indicated expression vectors and protein extracts were immunoprecipitated using Flag M2 beads. ( c ) Effects on BK channel ubiquitination by siRNA knockdown of individual CRL4A CRBN complex component. Cul4B is included as a negative control. The star indicates the nonspecific bands. ( d , e ) Effects on BK channel ubiquitination by ( d ) overexpression of CRBN(ΔMid), or ( e ) treating cells with thalidomide (50 μM) or MLN4924 (0.1 μM) for 6 h. Numerical band intensity was measured by NIH Image J and indicated on the figure. Thal, thalidomide. Full size image BK channels ubiquitinated by CRL4A CRBN are retained in the ER The ubiquitinated BK channels were not targeted for proteasome-dependent degradation, as knockdown or overexpression of various CRL4A CRBN subunits, or treating cells with proteasome inhibitor, had no obvious effects on the steady-state levels of the Slo1 protein ( Fig. 2c and Supplementary Figs 2a and 3 ). CRBN was reported to reduce the cell surface expression of BK channels [15] . We tested whether BK channel ubiquitination by CRL4A CRBN would alter BK channel subcellular localization. Using fluorescent confocal microscopy, we found that co-expression of CRBN, but not CRBN(ΔMid) mutant defective in binding CRL4A, redistributed BK channels from the cytoplasm and cell membrane to the juxtanuclear ER region in COS-7 ( Fig. 3a ) and HEK 293 cells ( Supplementary Fig. 4 ). Indirect immunofluorescence against extracellular BK channels in nonpermeabilized cells [27] confirmed that a dramatic decrease in BK channel expression at the cell membrane by CRBN expression requires the association of CRBN with CRL4A ( Fig. 3b ). This observation was further quantified using western blot analysis of the levels of cell surface BK channels that were biotinylated extracellularly ( Fig. 3c ). 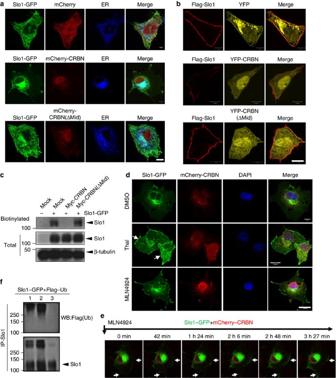Figure 3: CRL4ACRBNretains ubiquitinated BK channels in the ER and inhibits their surface expression in cultured cells. (a) Confocal fluorescent imaging of COS-7 cells transfected with Slo1-GFP and mCherry-CRBN or mCherry-CRBN(ΔMid). ER-Tracker was used to stain the ER. Scale bar, 10 μm. (b) Confocal imaging of cells transfected with N-terminally tagged Flag-Slo1 and YFP-CRBN or YFP-CRBN(ΔMid). The extracellular Flag epitope was visualized by indirect immunofluorescence under nonpermeabilized conditions. Scale bar, 10 μm. (c) Western blot analysis of the levels of extracellularly biotinylated BK channels in HEK 293 cells transfected with expression vectors of CRBN or CRBN(ΔMid). Cells were incubated with 1 mg ml−1Sulfo-NHS-SS-biotin solution. Surface biotinylated proteins were precipitated with streptavidin agrose resins. (d) Confocal imaging of COS-7 cells transfected with Slo1-GFP and mCherry-CRBN and treated with 50 μM thalidomide or 0.1 μM MLN4924 for 6 h. Scale bar, 20 μm. (e) Live imaging of COS-7 cells transfected with expression vectors for Slo1-GFP and mCherry-CRBN. Cells were monitored for 3 h 27 min and pictures were taken every 3 min after MLN4924 (0.1 μM) addition. White arrows indicate the distribution of GFP fusion BK channels on cell membranes. Scale bar, 10 μm. (f) HEK 293T cells were co-transfected with Slo1-GFP and Flag-Ub expression vectors. Membrane proteins were purified by biotinylation assay. Total and membrane proteins were subjected to Slo1 co-immunoprecipitation assays. (1) 1 × Total protein. (2) 2 × Total protein. (3) Membrane protein. Figure 3: CRL4A CRBN retains ubiquitinated BK channels in the ER and inhibits their surface expression in cultured cells. ( a ) Confocal fluorescent imaging of COS-7 cells transfected with Slo1-GFP and mCherry-CRBN or mCherry-CRBN(ΔMid). ER-Tracker was used to stain the ER. Scale bar, 10 μm. ( b ) Confocal imaging of cells transfected with N-terminally tagged Flag-Slo1 and YFP-CRBN or YFP-CRBN(ΔMid). The extracellular Flag epitope was visualized by indirect immunofluorescence under nonpermeabilized conditions. Scale bar, 10 μm. ( c ) Western blot analysis of the levels of extracellularly biotinylated BK channels in HEK 293 cells transfected with expression vectors of CRBN or CRBN(ΔMid). Cells were incubated with 1 mg ml −1 Sulfo-NHS-SS-biotin solution. Surface biotinylated proteins were precipitated with streptavidin agrose resins. ( d ) Confocal imaging of COS-7 cells transfected with Slo1-GFP and mCherry-CRBN and treated with 50 μM thalidomide or 0.1 μM MLN4924 for 6 h. Scale bar, 20 μm. ( e ) Live imaging of COS-7 cells transfected with expression vectors for Slo1-GFP and mCherry-CRBN. Cells were monitored for 3 h 27 min and pictures were taken every 3 min after MLN4924 (0.1 μM) addition. White arrows indicate the distribution of GFP fusion BK channels on cell membranes. Scale bar, 10 μm. ( f ) HEK 293T cells were co-transfected with Slo1-GFP and Flag-Ub expression vectors. Membrane proteins were purified by biotinylation assay. Total and membrane proteins were subjected to Slo1 co-immunoprecipitation assays. (1) 1 × Total protein. (2) 2 × Total protein. (3) Membrane protein. Full size image ER-retained BK channels were also released to the cell membrane by inhibition of CRL4A CRBN ligase activity with thalidomide or MLN4924 in COS-7 and HEK 293 cells that co-express BK channels and CRBN ( Fig. 3d and Supplementary Fig. 5 ). Time-lapse imaging of live cells treated with CRL4A CRBN inhibitors captured the dynamic process of time-dependent accumulation of BK channels at the cell surface ( Fig. 3e and Supplementary Movie 1 ). Quantification of the surface-expressed BK channels as a percentage of the total corroborates our conclusion that trafficking of BK channels from the ER to cell membrane requires enzymatically active CRL4A CRBN ligase ( Supplementary Fig. 6 ). To confirm that ubiquitinated BK channels fail to reach cell surface, Slo1 was immunoprecipitated from biotinylated proteins isolated from the plasma membrane and found to be barely ubiquitinated, in contrast to heavily ubiquitinated Slo1 in whole-cell lysates ( Fig. 3f ). We next explored the physiological relevance of CRL4A CRBN -mediated BK ubiquitination in primary neurons. Similar to COS-7 and HEK 293 cells, rat hippocampal neurons displayed ER-retained BK channel expression when co-expressed with CRBN ( Supplementary Fig. 7a ). However, co-expression of CRBN(ΔMid) led to a significant increase in BK channel expression in axons and dendrites ( Fig. 4a and Supplementary Fig. 7b ). Strikingly, neuronal surface expression was almost completely abolished by co-expression of CRBN, but not the mutant that fails to bind CRL4A ( Fig. 4b ). We further isolated hippocampal neurons [28] from mice with homozygous floxed DDB1 alleles ( DDB1 F/F ) [23] and deleted DDB1 by infecting these neurons with adenovirus expressing GFP-Cre. GFP + neurons, harbouring deleted DDB1, expressed abundant BK channels at cell surface, in contrast to barely any channels detected in GFP − neurons where CRL4A ligase is intact ( Fig. 4c ). These results indicate that CRL4A CRBN inhibits trafficking of BK channels to the neuronal surface. 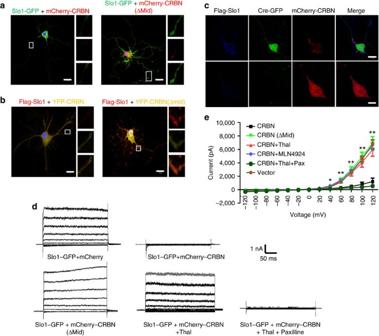Figure 4: Surface expression and electrophysiological function of BK channels are regulated by CRL4ACRBNE3 ligase. Confocal imaging of primary rat hippocampal neurons transfected with (a) Slo1-GFP and mCherry-CRBN or mCherry-CRBN(ΔMid) or (b) Flag-Slo1 and YFP-CRBN or YFP-CRBN(ΔMid). Surface expressed BK channels was labelled by Flag antibody under nonpermeabilized conditions. Scale bar, 20 μm. (c) Fluorescent imaging of primary hippocampal neurons dissected from P1DDB1F/Fmouse. These neurons were stained for extracellular Flag after being transfected with Flag-Slo1 and mCherry-CRBN and infected with adenovirus expressing Cre-GFP. Scale bar, 10 μm. (d) Currents of BK channels were recorded in whole-cell configuration in HEK 293 cells transfected with Slo1-GFP and mCherry-CRBN or mCherry-CRBN(ΔMid). Membrane potential of the cell was changed to a series of 400-mS step pulses from −120 to +120 mV in 20 mV increments. Cells were treated with thalidomide (50 μM) for 6 h before current recording. Further exploration was performed by adding paxilline (0.1 μM) at the time point before current recording. (e) Student’st-test was performed to analyse the currents from HEK 293 cells transfected with indicated expression vectors, with or without treatment of thalidomide, MLN4924 or Paxilline. The data represent the mean±s.e.m.*P<0.05, **P<0.01 (n=4–9 each group), Student’st-test. Figure 4: Surface expression and electrophysiological function of BK channels are regulated by CRL4A CRBN E3 ligase. Confocal imaging of primary rat hippocampal neurons transfected with ( a ) Slo1-GFP and mCherry-CRBN or mCherry-CRBN(ΔMid) or ( b ) Flag-Slo1 and YFP-CRBN or YFP-CRBN(ΔMid). Surface expressed BK channels was labelled by Flag antibody under nonpermeabilized conditions. Scale bar, 20 μm. ( c ) Fluorescent imaging of primary hippocampal neurons dissected from P1 DDB1 F/F mouse. These neurons were stained for extracellular Flag after being transfected with Flag-Slo1 and mCherry-CRBN and infected with adenovirus expressing Cre-GFP. Scale bar, 10 μm. ( d ) Currents of BK channels were recorded in whole-cell configuration in HEK 293 cells transfected with Slo1-GFP and mCherry-CRBN or mCherry-CRBN(ΔMid). Membrane potential of the cell was changed to a series of 400-mS step pulses from −120 to +120 mV in 20 mV increments. Cells were treated with thalidomide (50 μM) for 6 h before current recording. Further exploration was performed by adding paxilline (0.1 μM) at the time point before current recording. ( e ) Student’s t -test was performed to analyse the currents from HEK 293 cells transfected with indicated expression vectors, with or without treatment of thalidomide, MLN4924 or Paxilline. The data represent the mean±s.e.m. * P <0.05, ** P <0.01 ( n =4–9 each group), Student’s t -test. Full size image CRL4A CRBN inhibits the function of BK channels To determine the activity of BK channels that are released to the cell surface by inhibiting CRL4A CRBN , we recorded the ionic currents through BK channels by a whole-cell patch clamp method [29] . Representative traces of BK channel current, evoked by membrane depolarization, were recorded in HEK 293 cells ( Fig. 4d ). Co-expression of CRBN dramatically decreased BK channel current, consistent with reduced surface BK expression in these cells. However, treating these cells with thalidomide or MLN4924, or co-expression with CRBN(ΔMid) mutant rather than wild-type CRBN, restored BK channel current ( Fig. 4d ). Paxilline, a highly specific BK channel antagonist [30] , effectively blocked the channel activity that was restored in thalidomide-treated cells expressing BK and CRBN ( Fig. 4d,e ). These results suggest that BK channels released to the cell surface after CRL4A CRBN ligase inactivation are electrophysiologically functional. Inactivation of CRL4A CRBN induces epilepsy in mice Increased macroscopic current and neuronal excitability caused by a gain-of-function point mutation in BK channels can lead to generalized epilepsy in humans [11] , [31] . Since CRL4A CRBN inhibits surface expression of functional BK channels, we tested whether deregulation of this ubiquitin ligase in animals would cause epilepsy. We generated DDB1 F/F ;Camk2a-Cre mutant mice in which DDB1, an essential CRL4A ligase subunit, was conditionally ablated in postmitotic neurons of the hippocampus and cerebral cortex ( Supplementary Fig. 8 ) [32] . Unlike neuronal progenitor cells that undergo apoptosis after the loss of DDB1, DDB1-deficient neurons neither die or exhibit any DNA damage response nor accumulate established CRL4A ligase substrates including c-Jun, p21 or Cdt1 (data not shown). These mice develop normally without obvious growth or behavioural abnormality, except that some (10 out of 48), when aged 5 months or older, develop spontaneous seizures and/or convulsive death ( Fig. 5a ). 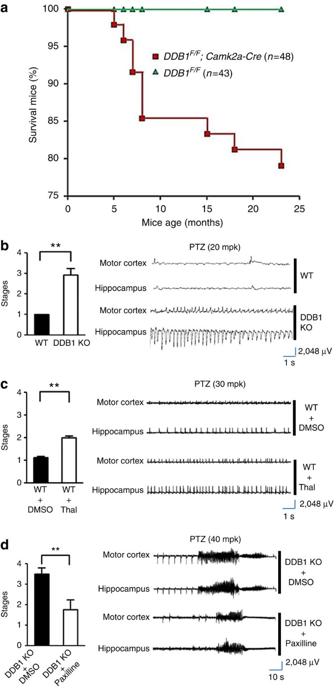Figure 5: Inactivation of CRL4ACRBNin mice leads to increased susceptibility to PTZ-induced epilepsy. (a) The survival curve ofDDB1F/F; Camk2α-Cremice. The death was induced by spontaneous seizure.n, total number of mice. (b–d) Scoring of seizure stages after PTZ injection (left) or representative EEG recording of one pair of mice. (b) Five-month-oldDDB1F/F; Camk2α-Cremice were injected i.p. with 20 mg kg−1PTZ, and taken to a new and clean cage where their behaviours were recorded on videotapes for 30 min. WT,DDB1F/Fmice. DDB1 KO,DDB1F/F; Camk2α-Cremice. Error bars indicate s.e.m. **P<0.01 (n=12 each group), Student’st-test. (c) Four-weeks-old C57/BL6 mice were divided into two groups and injected i.p. with 50 mg kg−1thalidomide or vehicle every 2 h for four times. Thirty minutes after last injection, mice were injected i.p. with 30 mg kg−1PTZ to induce epilepsy. **P<0.01 (n=19 each group), Student’st-test. (d) Five-month-oldDDB1F/F; Camk2α-Cremice injected i.p. with 2.2 μg kg−1paxilline or vehicle every 2 h for four times. Thirty minutes after last injection, mice were injected with 20 mg kg−1PTZ to induce epilepsy. **P<0.01 (n=4 each group), Student’st-test. Figure 5: Inactivation of CRL4A CRBN in mice leads to increased susceptibility to PTZ-induced epilepsy. ( a ) The survival curve of DDB1 F/F ; Camk2α-Cre mice. The death was induced by spontaneous seizure. n , total number of mice. ( b – d ) Scoring of seizure stages after PTZ injection (left) or representative EEG recording of one pair of mice. ( b ) Five-month-old DDB1 F/F ; Camk2α-Cre mice were injected i.p. with 20 mg kg −1 PTZ, and taken to a new and clean cage where their behaviours were recorded on videotapes for 30 min. WT, DDB1 F/F mice. DDB1 KO, DDB1 F/F ; Camk2α-Cre mice. Error bars indicate s.e.m. ** P <0.01 ( n =12 each group), Student’s t -test. ( c ) Four-weeks-old C57/BL6 mice were divided into two groups and injected i.p. with 50 mg kg −1 thalidomide or vehicle every 2 h for four times. Thirty minutes after last injection, mice were injected i.p. with 30 mg kg −1 PTZ to induce epilepsy. ** P <0.01 ( n =19 each group), Student’s t -test. ( d ) Five-month-old DDB1 F/F ; Camk2α-Cre mice injected i.p. with 2.2 μg kg −1 paxilline or vehicle every 2 h for four times. Thirty minutes after last injection, mice were injected with 20 mg kg −1 PTZ to induce epilepsy. ** P <0.01 ( n =4 each group), Student’s t -test. Full size image To systematically study the epileptiogenesis of these mice, their susceptibility to pentylenetetrazol (PTZ)-induced seizure was investigated [33] . Strikingly, a low-dose PTZ injection (20 mg kg −1 ) caused severe seizure, mostly at stages 3 and 4 accompanied with four to five recurrent seizures in 30 min, in all 5-month-old DDB1 F/F ;Camk2a-Cre mice, but had little effect on age- and sex-matched control DDB1 F/F mice ( Fig. 5b , Supplementary Fig. 9a for stage breakdown and Supplementary Movie 2 ). Electroencephalogram (EEG) recording confirmed that the hippocampus and motor cortex of mutant mice were far more excited than those of control mice ( Fig. 5b ). Consistent with the genetic model, treatment of wild-type mice with thalidomide sensitized animals to PTZ-induced seizure ( Fig. 5c and Supplementary Fig. 9b ), suggesting that CRL4A CRBN ubiquitin ligase activity is critical for suppressing the abnormal brain activity after chemical stimulation. Importantly, pretreatment of DDB1 F/F ;Camk2a-Cre mice with paxilline before PTZ injection mitigated the abnormally high excitation in the brain and reduced seizure severity ( Fig. 5d and Supplementary Fig. 9c ), demonstrating a direct contribution of activated BK channels to seizure onset in the DDB1 mutant mice. These in vivo data suggest that CRL4A CRBN ubiquitin ligase functions as a gatekeeper for epileptogenesis by suppressing the active BK channels. The ubiquitin system plays a major role in ER-associated degradation as well as endocytosis and lysosomal sorting of ion channels [34] . Here we reveal a new role of ubiquitin modification of ion channels in functional channel expression. In this case, CRL4A CRBN E3 ubiquitin ligase targets BK channels for ubiquitination on the ER and prevents ubiquitinated channels from trafficking to cell surface ( Supplementary Fig. 10a ). Impairing CRL4A CRBN activity would lead to the surface enrichment of BK channels and neuronal hyperexcitability, eventually exemplified by channelopathy such as epilepsy in patients ( Supplementary Fig. 10b ). In support, genetic ablation of DDB1, the subunits of CRL4A CRBN , in mice leads to enhanced susceptibility to seizure induction, which is also found in wild-type mice treated with pharmacological inhibition of the ligase. The seizures can be mitigated by pretreatment with paxilline, a BK channel inhibitor, suggesting a causal role of hyperactive BK channels in seizure onset in these mice. It remains to be determined whether deregulation of CRL4A CRBN E3 ligase activity could account for epilepsy of unknown aetiology. No mutations have yet been identified in Cul4A, DDB1 or CRBN in epilepsy patients. A nonsense mutation of CRBN is associated with non-syndromic learning deficit [21] ; therefore, it will be interesting to investigate whether the affected individuals ever suffer from seizure in their life time. It is also likely that activity of the CRL4A CRBN ligase might be downregulated to enhance BK activation during epileptogenesis. For example, Cullin family ubiquitin ligases are activated by nodulation [35] and inhibited by Cand1 (ref. 36 ); alterations of these regulators would achieve similar effects to those by mutations in CRL4A CRBN . In addition, mutations in BK channels have been identified by exon sequencing of samples from patients with idiopathic epilepsy [37] ; however,but whether these mutations affect CRL4A CRBN -mediated ubiquitination and membrane expression of BK channels have not been assessed. We established that pharmacological inhibition of CRL4A CRBN ligase activates BK channels. Thalidomide and its derivatives have been approved for treating leprosy and multiple myeloma. Efficacy of thalidomide family drugs positively correlates with high CRBN expression in multiple myeloma [38] , [39] . MLN4924 is in ongoing clinical trials for several types of haematopoietic cancer, inhibiting many more CRL enzymes than CRL4A CRBN . Treating patients chronically with these two compounds might lead to abnormal BK channel excitation and possible seizure incidents. Both gain- and loss-of-function BK channel mutations can generate neuronal hyperexcitability and contribute to variable epilepsy syndromes [40] . Drugs activating or inhibiting BK channels are being developed; however, their efficacy in treating or preventing seizures and epilepsy requires better understanding of BK channel regulation [40] , [41] . We reveal a previously unrecognized but important regulatory step of BK channel surface expression and activation. Our work points to an alternative therapeutic strategy to control BK channel activity by targeting CRL4A CRBN ubiquitin ligase in epilepsy patients. Mice The DDB1 F/F mice [23] were crossed with Camk2a-Cre transgenic mouse strains. The efficiency of DDB1 deletion specifically in the brain was confirmed with PCR reaction, Western blotting and immunohistochemistry using brain samples. Primers for the deleted allele, 5′-CCCACTTAAAGGACTGGTG-3′ and 5′-GGACAATGGAAACATAGGG-3′, were used to produce wild-type, 1,140-bp and deleted 320-bp fragments. All mice were maintained in a pathogen-free and temperature-controlled barrier facility with a 12-h-light/dark cycle in the centre for Experimental Animals at the Zhejiang University, Hangzhou, China. All animal experiments were conducted in accordance with protocols approved by the Committee for Animal Research of the Zhejiang University and conformed to the Guide for the Care and Use of Laboratory Animals (NIH publication no. 86-23, revised 1985). cDNA and plasmids DNA fragments corresponding to full-length, C-terminal, N-terminal, RCK1 or RCK2 domain of human Slo1 isoform b were amplified separately and subcloned into pXF6F expression vector from Xinhua Feng’s laboratory in the Zhejiang university between the Xba I and Hin dIII restriction sites, named as Slo1, Slo1(C), Slo1(N), Slo1(R1) and Slo1(R2), respectively. Full-length CRBN or CRBN(ΔMid) (deletion of the DDB1-binding domain) sequence were subcloned from pcDNA3.1-Flag-HA vector [17] and inserted into pXF4H, a gift from Xinhua Feng’s laboratoy, between the Xba I and Hin dIII sites. Full-length Slo1 was subcloned into the pEGFP-N1 vector using the Bgl II and Hin dIII restriction sites. CRBN and CRBN(ΔMid) sequences were also subcloned into pcDNA3-mCherry or pcDNA3-YFP vectors. The Flag-Slo1-HA expression vector was gifted from Michael J. Shipston (University of Edinburgh). Full-length DDB1 , Cul4A or Cul4B sequences were subcloned into pcDNA3.1(−)-Myc vector (also gifted from Zongping Xia’ laboratory in the Zhejiang university) between the Xba I and Hin dIII restriction sites. Antibodies Anti-BK channel (611248; BD Pharmingen), anti-Flag (F3165; Sigma), anti-HA (H6908; H3663; Sigma-Aldrich), anti-Myc (2272; Cell Signaling Technology), anti-Cul4A (A300-739A; Bethyl Laboratories), anti-Cul4B (2527-1; Epitomics), anti-DDB1 (37–6200; Invitrogen), anti-CRBN (H00051185-B01P; Abnova), anti-β-tubulin (32–2600; Invitrogen), anti-GFP (sc-8334; Santa Cruz Biotechnology) and anti-Flag M2 agarose (Sigma) were purchased and used according to the manufacturers’ recommendations. Cell culture and drug treatment HEK 293T cells, HEK 293 cells, HeLa cells and COS-7 cells obtained from the American Type Culture Collection (ATCC) were maintained at 37 °C in 5% CO 2 condition in DMEM (Gibco) supplemented with 10% fetal calf serum (Gibco) and 100 U ml −1 penicillin and streptomycin (Hyclone). Plasmids were transfected into HEK 293T, HEK 293 cells using PEI [42] . Thalidomide and MLN4924 were dissolved in DMSO, while drug treatment was performed by adding corresponding drug into medium 6 h before harvest. siRNA sequences and transfection The siRNA sequences for Cul4A were 5′-GAACUUCCGAGACAGACCUdTdT-3′ and 5′-GCAGAACUGAUCGCAAAGCAU-3′. The siRNA for Cul4B was 5-′AAGCCUAAAUUACCAGAAAdTdT-3′. The siRNA sequences for DDB1 were 5-′ACUAGAUCGCGAUAAUAAAdTdT and CCUGUUGAUUGCCAAAAACdTdT-3′. The siRNA sequence for CRBN was 5-′CAGCUUAUGUGAAUCCUCAUGGAUA-3′. siRNAs were transfected into HEK 293T cells using Lipofectamine 2000 (Invitrogen) according to the manufacturer’s instructions. Co-immunoprecipitation and western blot HEK 293T cells were transiently transfected with indicated plasmids and lysed in lysis buffer (150 mM NaCl, 1% NP-40, 50 mM Tris–HCl, pH 8.0, supplemented with complete set of protease inhibitors (Roche)). After centrifugation at 13,000 r.p.m. for 20 min, supernatants were subjected to immunoprecipitation by incubation with Flag M2 Affinity Gel (Sigma) or HA antibody followed by Protein A/G Agarose (GE Healthcare). The immunoprecipitates were separated with SDS–PAGE and analysed with western blot. Full-sized blots of cropped blots used in figures are included in Supplementary Fig. 11 . In vivo ubiquitination assay Ubiquitination assays were performed as described previously [43] . Briefly, Myc-Cul4A, Myc-Cul4B, Myc-DDB1, Flag-CRBN or siRNA for Cul4A, Cul4B, DDB1, CRBN were co-transfected with Flag-ubiquitin and HA-Slo1 in HEK 293T cells for 2 days. Cells were lysed in lysis buffer with a complete set of protease inhibitors. Slo1 was immunoprecipitated with HA antibody and analysed by immunoblotting with indicated antibodies. MG132 assay Myc-Cul4A, Myc-Cul4B, Myc-DDB1 were co-transfected with HA-Slo1(C) in HEK 293T cells. Cells were treated with 10 μM MG132 for 6 h. Lysates were analysed by Western blot. Cell surface biotinylation HEK 293 Cells were washed with ice-cold phosphate-buffered saline (PBS)++ (PBS with 1 mM CaCl 2 and 0.5 mM MgCl 2 ), labelled with 1 mg ml −1 sulfo-NHS-biotin (Pierce) in PBS++ for 30 min at 4 °C andthen quenched untreated biotin with cold 100 mM glycine for 10 min. After rinsing three times with PBS++, cells were lysed in lysis buffer (0.4% sodium deoxycholate, 63 mM EDTA, 50 mM Tris–HCl, pH 8.0, 1% Nonidet-40 and protease inhibitor mixture). Biotin-labelled cell surface proteins were isolated by incubating with streptavidin agarose resins (Thermo Scientific) at 4 °C overnight. Biotinylated BK channels were detected by immunoblotting using the BK channel antibody. Image acquisition and quantification HEK 293 or COS-7 cells were co-transfected with mCherry-CRBN (WT or ΔMid) and Slo1-GFP 24 h after seeding on 12-mm coverslips (pre-coated with Poly- L -Lysine). Twenty-four hours post-transfected cells were washed briefly in PBS and then fixed for 15 min at room temperature in 4% paraformaldehyde. After washing three times with PBS, cells were incubated with 4',6-diamidino-2-phenylindole reagent (1:1,000, Molecular Probes) to stain cell nuclei. Following three washes in PBS, coverslips were mounted on microscope slides using Mowiol. For staining the ER in live cells, ER-Tracker Blue-White DPX (Molecular Probes) was added to the culture medium at a dilution of 1:2,000. The cells were incubated for ~\n30 min under growth conditions and then continue to the following fixing steps. For chemical treatment experiments, 24-h post transfection, cells were treated with 50 μM thalidomide or 0.1 μM MLN4924 or dimethylsulphoxide for 6 h under growth conditions before fixation and immunofluorescence analysis. Confocal images were acquired on a Zeiss LSM710 laser scanning microscope (Karl Zeiss, Microimaging, GmbH, Germany) using a EC-plan-Neofluar × 40/1.3 or × 63/1.4 oil differential interference contrast M27 objective lens in multitracking mode to minimize channel cross-talk. All figure images were taken through the middle of the cell. For the fluorescence quantification, greyscale-inverted images and camera lucida drawing were generated using the Image J 1.60 software as described [44] . Background-subtracted total fluorescence intensity of the surface Flag and intracellular HA signal were measured and calculated to determine the surface/total ratios. All fluorescence intensity quantification values were reported as mean±s.e.m. Student’s t -test was performed to identify the statistically significant difference groups of two by using PRISM5 (GraphPad, San Diego, CA, USA). Live imaging COS-7 cells were co-transfected with mCherry-CRBN(WT) and Slo1-GFP 24 h after seeding into a 35-mm glass-bottom culture dish (Nest Biotechnology Co., Ltd, Jiangsu, China). At least 24 h after transfection, the cells were imaged. Images of live cells were acquired on an Olympus IX81 FV1000-XY confocal microscope (Imaging Core Facility, School of Medicine, Zhejiang University) and collected in sequential line mode. The exposure settings and gain of laser were kept constant and below the detected pixel saturation for each group of cells. All experiments were completed in triplicate ( n ≥3). Image analysis was performed with ImageJ ( http://rsb.info.nih.gov/ij ). Immunofluorescence Cell surface labelling of the N-terminal Flag epitope of BK channels in nonpermeabilized HeLa cells was performed as described [45] . Briefly, coverslips with transfected cells were washed with PBS and blocked in PBS containing 3% bovine serum albumin. A mouse monoclonal anti-Flag antibody (1:100 dilutions, M2, Sigma) was applied to cells for 1 h on ice. Alexa-594-conjugated anti-mouse IgG (1:1,000, Molecular Probes) was used as the secondary antibody. For the intracellular C-terminal HA epitope tag of Slo1 detection, the cells used above were subsequently washed three times and then fixed in 4% paraformaldehyde for 30 min, permeabilized with 0.1% Triton X-100 for 10 min and blocked with PBS containing 3% bovine serum albumin plus 0.05% Triton X-100 for 30 min. Anti-HA polyclonal rabbit antibody (1:100, 0.5 μg ml −1 , Zymed Laboratories Inc.) was added to cells and incubated for 1 h at room temperature. Dylight 405 AffiniPure Goat Anti-Rabbit IgG (H+L) (1:1,000, EarthOx, CA, USA) was used as the secondary antibody and the cells were washed three times before mounting. Primary neuron culture Mouse hippocampal primary neurons were prepared as previously described [28] . Briefly, pregnant female mice were killed when embryos were calculated to be at E16. Brain tissues were removed carefully from E16 embryos. The embryonic hippocampus was isolated gently under a dissecting microscope, rinsed in Hanks’ buffered saline solution, cut into small pieces, digested with Trypsin-EDTA, dissociated with a fire-polished glass pipette and centrifuged to separate undissociated tissue. Cells were then resuspended, plated on poly- L -lysine-coated 6-mm glass cover slides placed within six-well plates and maintained in neurobasal medium (Gibco, 21103-049) supplemented with 2% B27 (Gibco, 17504-044), 0.05 mM L -glutamine in an incubator at 37 °C with 5% CO 2 . Half the medium was replaced with fresh medium warmed to 37 °C every 3–4 days. Electrophysiology experiments HEK 293 cells were transfected with Slo1-GFP and mCherry, mCherry-CRBN or mCherry-CRBN(ΔMid) 24 h after seeding on 12-mm coverslips. Heat-polished borosilicate glass pipettes (2–5 M resistance) were filled with a pH 7.2 solution containing 140 mM KCl, 0.5 mM MgCl 2 , 1 mM EGTA, 5 mM ATP and 5 mM HEPES. Membrane potentials from −120 to +120 mV in 20-mV increments were applied to membrane patches for up to 400 ms using an Axopatch 200B voltage–current amplifier and the elicited currents were recorded using the pClamp 10.2 software. PTZ-induced seizure PTZ was injected i.p. at 20, 30 or 40 mpk to mice as indicated in each experiment. Treated mice were then placed in empty cages and recorded of their behaviour for 30 min. PTZ-induced seizure stages were classified into four stages [46] . Stage 1 was defined as hypoactivity, characterized by the animal being in the resting position with the abdomen fully touching the bottom of the cage. Stage 2 was defined as partial clonus, including that of the face, head or forelimbs. Stage 3 was defined as generalized clonus, consisting of rearing, falling and clonus of all four limbs and the tail. Stage 4 was defined as clonic–tonic (maximal) seizure, involving tonic hindlimb extension or death. Both stages 3 and 4 were considered as generalized seizures. Mice surgery and EEG recording Animals were anaesthetized with pentobarbital (50 mg kg −1 ) and mounted in a stereotaxic apparatus (SR-5N, Narishige, Japan). Electrodes were mounted in a stereotaxic apparatus (512600, Stoelting, USA) and implanted into right CA3 subfield of the ventral hippocampus (AP, −2.8; ML, −3.0; DV, −3.5) and right motor cortex (AP, 2.0; ML, −2.0; DV, −1.5). Reference and ground screws were placed in the bone over the cerebellum. All coordinates were measured in millimetre from bregma according to the atlas of Franklin and Paxinos (1997). The electrodes were made of twisted stainless steel teflon-coated wires (791500, diameter 0.125 mm, A.M. Systems, USA) insulated except at the tip 0.5 mm and the maximal tip separation was 0.5 mm. After 7–10 days of recovery, EEGs were recorded with band-pass filters spanning DC to 200 Hz and sampled at 2000 Hz by a digital amplifier (Synamps RT, Neuroscan System, USA) 15 min before PTZ injection. How to cite this article: Liu, J. et al. CRL4ACRBN E3 ubiquitin ligase restricts BK channel activity and prevents epileptogenesis. Nat. Commun. 5:3924 doi: 10.1038/ncomms4924 (2014).